Brief hearing loss disrupts binaural integration during two early critical periods of auditory cortex development Early binaural experience can recalibrate central auditory circuits that support spatial hearing. However, it is not known how binaural integration matures shortly after hearing onset or whether various developmental stages are differentially impacted by disruptions of normal binaural experience. Here we induce a brief, reversible unilateral conductive hearing loss (CHL) at several experimentally determined milestones in mouse primary auditory cortex (A1) development and characterize its effects ~1 week after normal hearing is restored. We find that CHL shapes A1 binaural selectivity during two early critical periods. CHL before P16 disrupts the normal coregistration of interaural frequency tuning, whereas CHL on P16, but not before or after, disrupts interaural level difference sensitivity contained in long-latency spikes. These data highlight an evolving plasticity in the developing auditory cortex that may relate to the aetiology of amblyaudia, a binaural hearing impairment associated with bouts of otitis media during human infancy. Perturbations of normal sensory experience during critical periods of cortical development can have specific and lasting effects on the organization of synapses, receptive fields, topographic maps and sensory-guided behaviours (for recent reviews see refs 1 , 2 ). Often, critical period regulation of a particular sensory representation coincides with a stage in normative development when its associated neural circuitry is most labile [3] . In the primary visual cortex, the effects of the eyelid suture are greatest several weeks after eye opening, when ipsilateral eye responses begin to rapidly mature [4] and the preferred stimulus orientation for inputs to each eye become increasingly well matched [5] . In the primary auditory cortex (A1) of altricial rodents, the effect of hearing loss on intracortical inhibition is greatest when inhibitory synapses are actively maturing [6] . Tonotopic map plasticity associated with pure tone rearing is limited to a 3-day window beginning at the onset of hearing, when tone-evoked response thresholds drop most precipitously [7] , synaptic excitation and inhibition are still uncorrelated [8] and dendritic spines on layer 4 thalamorecipient neurons are rapidly maturing [9] . By contrast, the effect of frequency-modulated sweep rearing on auditory directional tuning is greatest weeks later, when frequency-modulated sounds first begin to elicit high firing rates [10] . Temporarily disrupting hearing in one ear of young animals can negatively impact binaural selectivity in central auditory nuclei [11] , [12] , [13] , [14] , [15] , [16] , much like the effects of monocular deprivation on the development of coordinated binocular tuning in the visual cortex [2] . Unlike tonotopic map plasticity in the auditory cortex or ocular dominance plasticity in the visual cortex, the precise timing and organization of critical periods governing the experience-dependent maintenance of binaural integration in the developing auditory cortex are unknown. Moreover, it is not known how—or whether—these changes are aligned to the normal maturational time course for cortical binaural tuning. Thus, one of the aims for these experiments was to introduce a temporary hearing loss at precise time points suggested from a day-by-day analysis of normative binaural development in A1. Asymmetric conductive hearing loss (CHL) is quite common in human infants with otitis media [17] . Affected individuals are at greater risk to experience a constellation of brain-based binaural hearing impairments in later life, collectively known as amblyaudia (named after its visual analogue, amblyopia (for review see ref. 18 )). However, developmental studies of temporary CHL in animal models generally involve recording immediately following extended periods of severe CHL rather than simulating the more enduring effects of the transient, moderate-intensity CHL that can accompany otitis media [17] . Therefore, a second goal of these studies was to determine whether mimicking a naturally occurring CHL at empirically defined developmental milestones is associated with specific neuronal deficits in binaural integration. To address these aims, we tracked the day-by-day maturation of A1 sound representations over the first week of hearing in mouse pups. We noted abrupt shifts in monaural response threshold and preferred frequency tuning between P11 and P14 followed by a more gradual maturation of ipsilateral interaural level difference (ILD) sensitivity contained in long-latency spikes that was maximally pronounced at P15–P16. To test the hypothesis that the stepwise time course of normative maturation would correspond to distinct points in development when each feature was specifically vulnerable to the effects of degraded binaural experience, we introduced a brief, reversible monaural CHL at P12, P16 or P20. We found that disrupting binaural experience at P12 interfered with the normal coregistration of frequency-receptive fields between the contralateral and ipsilateral ears, whereas the same manipulation at P16 primarily affected cortical ILD sensitivity. These findings highlight a sequence of brief developmental windows occurring shortly after hearing onset that regulate the specific and lasting influence of binaural experience on the cortical representation of sound features underlying spatial hearing. Defining the onset of hearing The maturation of cortical sound representations was characterized on a day-by-day basis for 1 week after the onset of hearing. The analysis was based on recordings from 1,262 A1 units in 35 CBA/CaJ mice. The onset of hearing was operationally defined as P10, as it was the earliest age when a contiguous monaural frequency response area (FRA) could be delineated from the anaesthetized cortex using airborne tone bursts ≤90 dB sound pressure level (SPL) (albeit, in only 3/64 recordings sites from one of the three P10 pups tested). This does not set an absolute lower bound on the onset of hearing in all mice, as measurements in different strains or with different functional markers of hearing could provide different results. However, P10 or P11 is the age at which the ear canal first opens in several mouse strains, Preyer’s reflex is first evident and sound-evoked activity is first observed in the auditory nerve and inferior colliculus, making it a reasonable estimate [19] , [20] , [21] . Development of monaural sound representations Monaural FRAs exhibit a series of profound changes during the first week of hearing ( Fig. 1a ). At the onset of hearing, contralateral and ipsilateral best frequencies (BFs) were predominantly found between 10 and 22 kHz, frequencies that fall within the most sensitive region of the CBA mouse audiogram [22] . Beginning at P14, contralateral and ipsilateral BFs were observed at progressively more eccentric sound frequencies until they reached an adult-like distribution by P16 or P17 ( Fig. 1b ). Contralateral and ipsilateral minimum response thresholds also decreased significantly during the initial days of hearing, reaching approximately adult-like levels by P15 (one-way analysis of variances (ANOVAs), F >120.43, P <1 × 10 −6 for both contralateral ( n =964) and ipsilateral ( n =684) response measurements, Fig. 1c ). 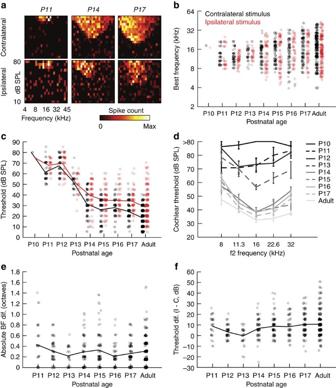Figure 1: Rapid maturation of monaural response properties in A1 is associated with concurrent changes in cochlear sensitivity. (a) Representative contralateral and ipsilateral FRAs recorded from A1 on P11, P14 and P17. (b,c) Rapid expansion of BF (b) and drop in threshold (c) of contralateral (black) and ipsilateral (red) FRAs measured from 1,001 units in 35 mice. (d) Minimum sound levels sufficient to elicit a measurable DPOAE at five test frequencies.N=56 ears, values represent mean±s.e.m. DPOAEs are based on outer hair cell receptor currents that can be measured as sound level changes in the ear canal. (e,f) Neither the absolute difference between contralateral and ipsilateral BFs (e) nor the contralateral bias in minimum response threshold (f) were greatly changed over the first week of hearing. C, contralateral; I, ipsilateral; dif., difference. Lines represent mean values at each age. Each data point is one recording site. A slight random jitter is imposed on all data points to visually distinguish identical values in the scatterplots. Figure 1: Rapid maturation of monaural response properties in A1 is associated with concurrent changes in cochlear sensitivity. ( a ) Representative contralateral and ipsilateral FRAs recorded from A1 on P11, P14 and P17. ( b , c ) Rapid expansion of BF ( b ) and drop in threshold ( c ) of contralateral (black) and ipsilateral (red) FRAs measured from 1,001 units in 35 mice. ( d ) Minimum sound levels sufficient to elicit a measurable DPOAE at five test frequencies. N =56 ears, values represent mean±s.e.m. DPOAEs are based on outer hair cell receptor currents that can be measured as sound level changes in the ear canal. ( e , f ) Neither the absolute difference between contralateral and ipsilateral BFs ( e ) nor the contralateral bias in minimum response threshold ( f ) were greatly changed over the first week of hearing. C, contralateral; I, ipsilateral; dif., difference. Lines represent mean values at each age. Each data point is one recording site. A slight random jitter is imposed on all data points to visually distinguish identical values in the scatterplots. Full size image The rapid maturation of cortical response properties in the first days after hearing onset could reflect neurodevelopmental changes in the central auditory system and/or the auditory periphery. To estimate postnatal changes in cochlear sensitivity, we measured the outer hair cell function via distortion product otoacoustic emissions (DPOAEs), a bioacoustic signal that is based upon sound-evoked changes in hair cell receptor potentials that can be measured as sound pressure changes in the ear canal [23] . In so doing, it was evident that both the change in A1 response thresholds and the increasing range of BF tuning between P10 and P14 occurred in parallel with commensurate changes in cochlear sensitivity (ANOVA, main effect for DPOAE threshold changes by age and age × frequency interaction term n =56 ears, F =77.38 and 3.52, respectively, P <1 × 10 −6 for both comparisons; Fig. 1d ). The contribution of peripheral maturation to developmental changes in A1 threshold and frequency sensitivity can be accounted for if one assumes that peripheral maturation is symmetrical; namely, whatever developmental processes are unfolding in the left ear are also unfolding in the right ear. In this scenario, the intearaual difference in various response features would remain constant, despite ongoing cochlear maturation. Alternatively, peripheral development could accompany changes in CNS circuits tuned to interaural response features. This could result in developmental changes in both monaural and interaural response properties. To address these possibilities, we analysed developmental changes in the interaural relationship between various response features for units with contralateral and ipsilateral receptive fields (71% of all recording sites). We found that interaural BFs deviated by ~0.25 octaves throughout the first week of hearing (one-way ANOVA, n =707, F =1.54, P =0.15; Fig. 1e ). This suggested that the rapid increase in the range of preferred frequency tuning noted in Fig. 1b can be primarily attributed to postnatal changes in cochlear development, as has been suggested previously [24] , [25] . The interaural threshold difference increased slightly but significantly across the ages tested (one-way ANOVA, n =707, F =8.49, P <1 × 10 −6 ; Fig. 1f ). Although this supports a previous description of increasing contralateral sensitivity bias across an early period of hearing in the ferret cortex [26] , the increase in the interaural threshold difference is far less than the change in overall response threshold ( Fig. 1c ). Collectively, these findings suggest that many changes in monaural threshold and frequency tuning can be ascribed to cochlear development. Despite its provenance, the fact remains that the sensitivity and frequency range of sound-evoked spiking changes dramatically between P11 and P14 in A1. The timing of this abrupt change in cortical spiking patterns may predict the timing of a critical period window for experience-dependent influences on coordinated interaural frequency tuning. Monaural deprivation disrupts receptive field balance To test this hypothesis, we developed a new approach to temporarily degrade auditory inputs to one ear during brief windows of postnatal development. This was achieved by injecting a thermoreversible poloxamer hydrogel into the middle ear cavity, which simulated a temporary bout of asymmetric CHL that can accompany otitis media in human infants ( Fig. 2a ). Poloxamers offer the advantage of remaining liquid when injected in the middle ear at a cool temperature, then rapidly transition to a gel as they warm to body temperature and, finally, spontaneously dissolve through hydrolysis several days later. Intratympanic poloxamer injections circumvent some of the challenges associated with using ear plugs in very young animals, such as permanent stenosis of the ear canal and degradation of the tympanic membrane [27] . It also provides an alternative to surgically ligating the ear canal, which is disadvantaged by the fact that normal hearing thresholds can only be restored by an invasive surgery on the ligated ear, thereby necessitating that the neurophysiology experiment take place within minutes or hours after hearing is restored. By tracking day-to-day changes in auditory brainstem response (ABR) in mice injected with poloxamer at P16 and P17 ( n =14) or age-matched control mice ( n =9), we determined that poloxamer injections induced a significant elevation of ABR wave 1 threshold for 5 days at 8 kHz ( Fig. 2b ), 6 days at 16 kHz ( Fig. 2c ) and 7–13 days at 32 kHz ( Fig. 2d ). We also confirmed that the ABR threshold shift was fully resolved before our cortical neurophysiology experiments 14–15 days after the initial poloxamer injection (that is ~1 week after normal hearing was restored, Fig. 2e ). 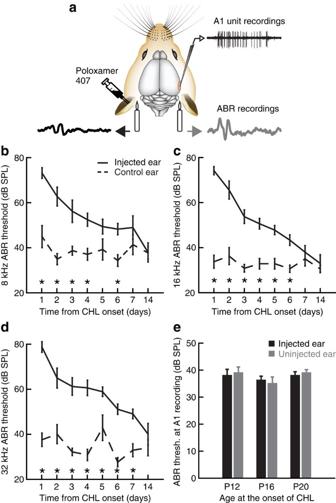Figure 2: Intratympanic poloxamer injections create a short-term and fully reversible mild CHL. (a) Reversible CHL was created by injecting a solution of Poloxamer 407, a thermoreversible hydrogel, into the middle ear space of young mice. Injections were made on two consecutive days into the left ear. Unit recordings were made in the right A1, contralateral to the injected ear. (b–d) Minimum response threshold for ABR wave 1 elicited with 8 (b), 16 (c) or 32 kHz (d) tone bursts delivered to the left ear. Thresholds are plotted relative to day of the first poloxamer injection on P16 (solid lines,n=14) or from age-matched control mice (dashed lines,n=9). (e) ABR threshold was measured at 16 kHz from left injected ear (black) and the right uninjected ear (grey) in poloxamer-injected mice. Measurements were taken immediately before A1 recordings, 14 days after an initial poloxamer injection at P12 (n=5), P16 (n=4) or P20 (n=5). All values represent mean±s.e.m. Asterisks indicate significant differences between poloxamer and control threshold values based on ANOVApost-hocpairwise comparisons (P<0.05). Figure 2: Intratympanic poloxamer injections create a short-term and fully reversible mild CHL. ( a ) Reversible CHL was created by injecting a solution of Poloxamer 407, a thermoreversible hydrogel, into the middle ear space of young mice. Injections were made on two consecutive days into the left ear. Unit recordings were made in the right A1, contralateral to the injected ear. ( b – d ) Minimum response threshold for ABR wave 1 elicited with 8 ( b ), 16 ( c ) or 32 kHz ( d ) tone bursts delivered to the left ear. Thresholds are plotted relative to day of the first poloxamer injection on P16 (solid lines, n =14) or from age-matched control mice (dashed lines, n =9). ( e ) ABR threshold was measured at 16 kHz from left injected ear (black) and the right uninjected ear (grey) in poloxamer-injected mice. Measurements were taken immediately before A1 recordings, 14 days after an initial poloxamer injection at P12 ( n =5), P16 ( n =4) or P20 ( n =5). All values represent mean±s.e.m. Asterisks indicate significant differences between poloxamer and control threshold values based on ANOVA post-hoc pairwise comparisons ( P <0.05). Full size image To compare the effects of temporary unilateral hearing loss on the coordinated development of interaural frequency tuning, recordings were made from A1 in the right hemisphere of mice 2 weeks after poloxamer injection into the left middle ear cavity on P12 (CHL12), P16 (CHL16) or P20 (CHL20), and also from mice that underwent a sham procedure at one of these ages. Unless otherwise indicated, descriptive statistics are provided as mean±s.e.m. P -values for all statistical tests reported below are based on an ANOVA followed up with pairwise contrasts that were adjusted for multiple comparisons with the Bonferroni method. In sham-operated juvenile mice, as was previously described in naive adult mice, contralateral FRA thresholds were 5 dB lower on average than ipsilateral FRA thresholds (21.1±0.94 versus 25.9±1.25 dB, Fig. 1f and Fig. 3a,b ). A double dissociation was observed for tone sensitivity in CHL12 mice, such that thresholds for the developmentally deprived contralateral ear were significantly elevated (26.04±0.77 dB, ANOVA post-hoc comparison, n =212, P <0.005), whereas sensitivity to the non-deprived ipsilateral ear was significantly enhanced relative to shams (20.0±0.79 dB, ANOVA post-hoc comparison, n =212, P <0.0005; Fig. 3a,b ). CHL initiated at P16 was associated with a significant elevation in the contralateral deprived ear threshold compared with sham (25.28±0.9 dB, ANOVA post-hoc comparison, n =204, P <0.05) but no change in ipsilateral threshold (24.76±0.96 dB, ANOVA post-hoc comparison, n =204, P >0.5). Contralateral and ipsilateral FRA thresholds from CHL20 recordings were not different than sham controls (22.46±0.83 and 27.46±0.84 dB for contralateral and ipsilateral, respectively, ANOVA post-hoc comparison, n =195, P >0.9 for both). The spontaneous firing rate was also elevated when CHL was initiated at P12 compared with sham, but not at any other age (18.64±0.85 versus 12.71±0.81 spikes per s, ANOVA post-hoc comparison, n =305, P <1 × 10 −6 , Fig. 3c ). 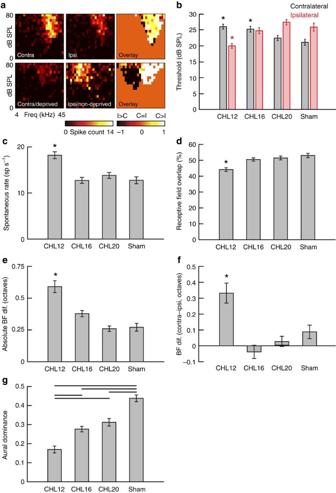Figure 3: An early critical period for the disruptive effect of transient unilateral hearing loss on interaural receptive field alignment. (a) Representative contralateral and ipsilateral FRAs recorded from A1 of mice that received a sham procedure (top) or a poloxamer injection to the contralateral ear on P12 (bottom). All recordings are made 14–15 days following the initial poloxamer injection or sham procedure. For purposes of direct comparison, the monaural FRA colour scale is mapped to the same range of firing rates rather than normalizing individually. Panels to the right represent the ratio of firing rates for each point within the union of the contralateral and ipsilateral FRAs. (b) Contralateral (black) and ipsilateral (red) FRA thresholds. (c) Spontaneous firing rate measured during the 100-ms period preceding tone onset. (d) The percentage of tone combinations contained in both contralateral and ipsilateral FRAs (the intersection) relative to all tone combinations contained in the contralateral and ipsilateral FRAs combined (the union). (e) Absolute difference in BF measured from the contralateral and ipsilateral FRAs. (f) Increased BF disparity in CHL12 group reflects a systematic high-frequency shift in contralateral versus ipsilateral BFs. Asterisk indicates a significant difference based on a paired Student’st-test (P<0.005). (g) Mean ratio of contralateral versus ipsilateral firing rates from tone combinations within the union of both FRAs. More positive values indicate greater contralateral dominance. All values represent mean±s.e.m. dif., difference. Sample size: CHL12 (n=163 (total units)/135 (units with bilateral FRAs) from 6 mice), CHL16 (n=159/127 units from 5 mice), CHL20 (n=149/127 units from 5 mice) and sham-operated controls (n=142/77 units from 5 mice). Asterisks and horizontal lines indicate significant differences relative to the sham group or associated pair, respectively, according to ANOVApost-hocpairwise statistics adjusted for multiple comparisons (P<0.05). Figure 3: An early critical period for the disruptive effect of transient unilateral hearing loss on interaural receptive field alignment. ( a ) Representative contralateral and ipsilateral FRAs recorded from A1 of mice that received a sham procedure (top) or a poloxamer injection to the contralateral ear on P12 (bottom). All recordings are made 14–15 days following the initial poloxamer injection or sham procedure. For purposes of direct comparison, the monaural FRA colour scale is mapped to the same range of firing rates rather than normalizing individually. Panels to the right represent the ratio of firing rates for each point within the union of the contralateral and ipsilateral FRAs. ( b ) Contralateral (black) and ipsilateral (red) FRA thresholds. ( c ) Spontaneous firing rate measured during the 100-ms period preceding tone onset. ( d ) The percentage of tone combinations contained in both contralateral and ipsilateral FRAs (the intersection) relative to all tone combinations contained in the contralateral and ipsilateral FRAs combined (the union). ( e ) Absolute difference in BF measured from the contralateral and ipsilateral FRAs. ( f ) Increased BF disparity in CHL12 group reflects a systematic high-frequency shift in contralateral versus ipsilateral BFs. Asterisk indicates a significant difference based on a paired Student’s t -test ( P <0.005). ( g ) Mean ratio of contralateral versus ipsilateral firing rates from tone combinations within the union of both FRAs. More positive values indicate greater contralateral dominance. All values represent mean±s.e.m. dif., difference. Sample size: CHL12 ( n =163 (total units)/135 (units with bilateral FRAs) from 6 mice), CHL16 ( n =159/127 units from 5 mice), CHL20 ( n =149/127 units from 5 mice) and sham-operated controls ( n =142/77 units from 5 mice). Asterisks and horizontal lines indicate significant differences relative to the sham group or associated pair, respectively, according to ANOVA post-hoc pairwise statistics adjusted for multiple comparisons ( P <0.05). Full size image In addition to a bidirectional adjustment in sensitivity, we also observed that contralateral and ipsilateral receptive fields, which were precisely coregistered for frequency preference even at the onset of hearing ( Fig. 1e ), had slipped out of alignment when CHL was initiated at P12 ( Fig. 3a ). Quantitative analysis confirmed that the percentage of overlapping points in contralateral and ipsilateral FRAs was significantly reduced (53±1% versus 44±1%; ANOVA post-hoc comparison, n =212, P <5 × 10 −5 , Fig. 3d ) and that BFs were approximately twice as far apart in CHL12 recordings (0.59±0.05 versus 0.27±0.03 octaves; ANOVA post-hoc comparison, n =212, P <1 × 10 −6 ), but were not different than sham recordings in CHL16 or CHL20 conditions (ANOVA post-hoc comparisons, n =204 and n =195, respectively, P >0.24 for all comparisons, Fig. 3e ). The increase in absolute BF difference in CHL12 recordings was attributed to a systematic high-frequency shift in contralateral compared with ipsilateral BF, as has also been reported shortly after mild sensorineural hearing loss in primates [28] (0.33±0.06 octaves, paired Student’s t -test, n =212, P <0.005, Fig. 3f ). As a final comparison of interaural dominance, the average ratio of firing rates for all points within the union of the contralateral and ipsilateral FRAs were compared, where the degree of positivity is commensurate with the degree of contralateral bias in evoked firing rate (right-most column in Fig. 3a ). The contralateral bias measured from all three deprivation ages was reduced compared with shams (CHL12, 0.16±0.02; CHL16, 0.28±0.01; CHL20, 0.31±0.02; Sham, 0.44±0.02; ANOVA post-hoc comparisons, n =212, 204 and 195, respectively, P <5 × 10 −5 for all comparisons), yet the decrease was significantly greater in CHL12 recordings compared with either CHL16 or CHL20 (ANOVA post-hoc comparisons, n =262, P <5 × 10 −5 for both, Fig. 3g ), matching an earlier description that A1 aural dominance plasticity effects subsequent to unilateral CHL are observed into adulthood but are most pronounced when asymmetric hearing loss is initiated shortly after hearing onset [15] . Other than this graded change in contralateral response bias, most aspects of interaural frequency tuning were only modified by CHL initiated at P12, the age in normative development when response thresholds and preferred frequency tuning were poised to change most abruptly. Development of ILD selectivity The position of a sound source along the horizon is encoded centrally by neurons sensitive to differences in the loudness or timing of sounds arriving at each ear. Therefore, the development of binaural integration must predominantly reflect maturation of central binaural circuits. In mammals such as rats and mice, which have small head circumferences, high-frequency hearing ranges and a virtually non-existent medial superior olivary nucleus, ILD contributes far more actionable information for sound localization than interaural time differences [29] , [30] . In response to brief dichotic sounds that vary in ILD or spatial location, most cortical units exhibit robust responses to contralateral stimuli and suppressed responses to ipsilateral stimuli [31] , [32] , [33] , [34] . Thus, most auditory cortex units, whether recorded in adulthood or shortly after hearing onset have been described as ‘ EI ’, a categorical label denoting a net excitatory ( E ) input from the contralateral ear and a net inhibitory ( I ) input from the ipsilateral ear [35] , [36] . Several studies have demonstrated that the cortical representation of binaural sound level is considerably more nuanced than the categorical label ‘ EI ’ would suggest [34] . In fact, spikes evoked by dichotic sounds may contain information about multiple binaural level combinations, and the representational salience of disparate stimulus features can be wax and wane on distinct time scales within the overall stimulus-evoked response period [37] , [38] , [39] . To further explore the possibility that spikes associated with contralateral versus ipsilateral ILD combinations may occur in distinct periods within the overall stimulus-evoked response, and the maturation of this dichotomous ILD sensitivity may be regulated on distinct developmental time scales, we adopted an unbiased brute force search algorithm to identify and separately analyse the post-stimulus time periods associated with the strongest differential sensitivity to contralateral versus ipsilateral ILD combinations. At the onset of hearing, short-latency spikes were strongly tuned for contralateral ILDs in a manner consistent with the EI designation previously described in infant and adult A1 units ( Fig. 4a ). Moreover, at the onset of hearing, even the optimal temporal windowing failed to capture any selectivity for ipsilateral ILDs ( Fig. 4b ). Recordings made from mice just a few days older revealed a similar short-latency response period containing contralateral ILD sensitivity ( Fig. 4c ), but in contrast to recordings made at P11 clear sensitivity for ipsilateral ILDs was present at longer latencies ( Fig. 4d ). 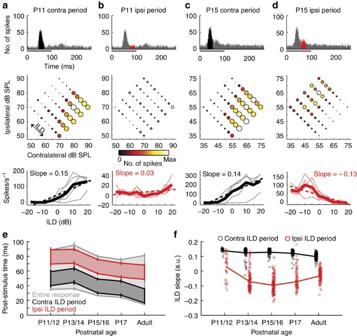Figure 4: Maturation of ILD sensitivity during the first week of hearing. (a–d) Top rows: post-stimulus time histograms of spikes recorded from an A1 units at P11 (a,b) or P15 (c,d) following a 100-ms dichotic white noise burst (horizontal bar). Histogram colouring depicts timing of spikes that showed the strongest differential sensitivity to contralateral ILDs (black) and ipsilateral ILDs (red). Middle rows: bubble plots present firing rate as a function of ILD across five mean binaural levels based on the spike windowing shown above. Heat map is scaled to the normalized firing rate within each time window, whereas circle diameter is normalized to the maximum firing rate across both time windows. Bottom rows: faint lines represent firing rate changes across ILD at each of five binaural levels between threshold and 20 dB>threshold. Thick and dashed lines represent the mean ILD-rate function and its linear fit, respectively. Numerical slope of the fit line (the ILD slope value) is provided. (e) Mean±s.e.m. onset (lower value) and offset (higher value) of the entire stimulus-evoked response period (light gray), optimal contralateral (dark grey) and ipsilateral (red) ILD periods. (f) ILD slope values across all ages (n=39 units from 6 P11/P12 mice,n=148 form 7 P13/14 mice,n=180 from 6 P15/16 mice,n=96 from 3 P17 mice andn=147 from 9 adult mice). Positive and negative slope values indicate a preference for contralateral and ipsilateral ILDs, respectively, for spikes contained within the optimal contralateral (black) or ipsilateral (red) ILD response periods. Lines represent mean values at each age. Each data point is one recording site. A slight random jitter is imposed on all data points to visually distinguish identical values in the scatterplots. Figure 4: Maturation of ILD sensitivity during the first week of hearing. ( a – d ) Top rows: post-stimulus time histograms of spikes recorded from an A1 units at P11 ( a , b ) or P15 ( c , d ) following a 100-ms dichotic white noise burst (horizontal bar). Histogram colouring depicts timing of spikes that showed the strongest differential sensitivity to contralateral ILDs (black) and ipsilateral ILDs (red). Middle rows: bubble plots present firing rate as a function of ILD across five mean binaural levels based on the spike windowing shown above. Heat map is scaled to the normalized firing rate within each time window, whereas circle diameter is normalized to the maximum firing rate across both time windows. Bottom rows: faint lines represent firing rate changes across ILD at each of five binaural levels between threshold and 20 dB>threshold. Thick and dashed lines represent the mean ILD-rate function and its linear fit, respectively. Numerical slope of the fit line (the ILD slope value) is provided. ( e ) Mean±s.e.m. onset (lower value) and offset (higher value) of the entire stimulus-evoked response period (light gray), optimal contralateral (dark grey) and ipsilateral (red) ILD periods. ( f ) ILD slope values across all ages ( n =39 units from 6 P11/P12 mice, n =148 form 7 P13/14 mice, n =180 from 6 P15/16 mice, n =96 from 3 P17 mice and n =147 from 9 adult mice). Positive and negative slope values indicate a preference for contralateral and ipsilateral ILDs, respectively, for spikes contained within the optimal contralateral (black) or ipsilateral (red) ILD response periods. Lines represent mean values at each age. Each data point is one recording site. A slight random jitter is imposed on all data points to visually distinguish identical values in the scatterplots. Full size image Looking across the developmental ages studied here, the optimal period for contralateral ILD sensitivity occurred significantly earlier within the overall response period than the optimal ipsilateral ILD period (mixed-design ANOVA, n =610, F >1,660, P <1 × 10 −6 for both onset and offset main effects; Fig. 4e ). ILD sensitivity changed significantly over the early period of hearing, although in different ways and at different rates within the early- and late-occurring response windows. At the onset of hearing, A1 binaural tuning was essentially purely EI . Contralateral ILD sensitivity was relatively constant across age, although ILD slopes flattened somewhat between P17 and adulthood, resulting in a subtle but significant reduction in the short-latency contralateral ILD slope across development (one-way ANOVA, n =610, F =56.25, P <1 × 10 −6 ; black symbols in Fig. 4f ). Conversely, negatively sloped ipsilateral ILD sensitivity was rarely observed at the onset of hearing ( Fig. 4b , bottom row, and Fig. 4f , red symbols). However, negative slope values indicating separable ipsilateral ILD sensitivity in long-latency spikes emerged several days later, became maximally defined at P15 and P16 and returned to an intermediate, although still clearly separable, state in adulthood (one-way ANOVA, n =610, F =47.0, P <1 × 10 −6 ; Fig. 4f ). Transient hearing loss weakens cortical ILD sensitivity The normative course of ILD maturation in A1 suggested that contralateral ILD sensitivity was roughly adult-like at the onset of hearing, whereas the weaker, temporally delayed response to ipsilateral ILDs was effectively absent at the onset of hearing and continued to change significantly through P17. Working off the premise that the developmental windows for experience-dependent reorganization would coincide with the period of greatest change in normative development, we hypothesized that contralateral ILD sensitivity would be only weakly affected by CHL. By contrast, the effect of CHL on ipsilateral ILD sensitivity would be both greater in magnitude and developmentally delayed compared with both contralateral ILD and interaural FRA changes ( Fig. 3 ). The example recordings shown in Fig. 5a–c confirm that transient unilateral CHL disrupted distinct aspects of binaural integration depending upon whether it began at P12 or P16. Compared with sham recordings ( Fig. 5a ), CHL at P12 was associated with slightly reduced contralateral ILD slope values (0.08±0.01 versus 0.1±0.01, ANOVA post-hoc comparison, n =292, P <1 × 10 −6 ) but comparable sensitivity to ipsilateral ILDs (−0.03±0.01 versus −0.03±0.01, ANOVA post-hoc comparison, n =292, P =1.0; Fig. 5b,d ). The opposite pattern was noted in CHL16 recordings; namely, contralateral ILD sensitivity was similar to controls (0.1±0.01, ANOVA post-hoc comparison, n =370, P =1.0), yet ipsilateral ILD sensitivity was abolished (0.0±0.01, ANOVA post-hoc comparison, n =370, P <1 × 10 −6 ; Figs. 5c,d ). These same trends were noted in the best ILD, defined as the ILD combination that yielded the highest average firing rate. In CHL12 recordings, the preferred ILD within the contralateral period was shifted closer to zero than shams (13±0.77 versus 17.08±0.46 dB, ANOVA post-hoc comparison, n =292, P <1 × 5 −5 ), yet the best ipsilateral ILD was equivalent (−6.37±0.92 versus −4.78±1.03 dB, ANOVA post-hoc comparison, n =292, P =1.0; Fig. 5e ). Conversely, initiating hearing loss at P16 had no effect on the preferred ILD in the contralateral period (16.79±0.36 dB, ANOVA post-hoc comparison, n =370, P =1.0), yet the best ILDs from the ipsilateral response window were significantly more contralaterally biased than in sham recordings (4.23±1.12 dB, ANOVA post-hoc comparison, n =370, P <1 × 10 −6 ; Fig. 5e ). Initiating transient CHL at P20 had no effect on the ILD slope or best ILD values derived from either of the response windows when compared with sham controls (ANOVA post-hoc comparisons, n =260, P >0.16 for all comparisons; Fig. 5d,e ). Systematic differences in the timing of the contralateral (23–30 ms post-stimulus onset across all groups) or ipsilateral ILD windows (51–56 ms post-stimulus onset across all groups) were not observed. 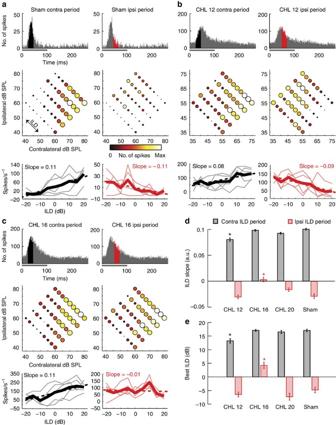Figure 5: Temporary CHL disrupts short- and long-latency ILD sensitivity at distinct ages during the first week of hearing. (a–c), PSTHs (top row), binaural interaction matrices (middle row) and ILD-rate functions (bottom row) derived from the optimal contralateral and ipsilateral ILD response periods (black and red, respectively) from representative A1 recording sites in sham and poloxamer-injected mice. All plotting conventions are identical to those used inFig. 4. Note the double dissociation between disruptions of short-latency contralateral ILD sensitivity in the CHL12 unit (b) and long-latency ipsilateral ILD sensitivity in the CHL16 unit (c) compared with sham (a). (d) Slope of the linear fits applied to ILD-rate functions derived from the early contralateral (black) and late ipsilateral (red) ILD response windows (n=127 sham units from 5 mice, 165 CHL12 units from 6 mice, 143 CHL16 units from 5 mice and 117 CHL20 units from 5 mice). (e) ILD associated with the highest firing rate (that is, the best ILD) based on the contralateral (black) versus ipsilateral (red) ILD response windows. All values represent mean±s.e.m. Asterisks indicate a significant difference relative to the sham group with an ANOVA after correcting for multiple comparisons (P<0.05). Figure 5: Temporary CHL disrupts short- and long-latency ILD sensitivity at distinct ages during the first week of hearing. ( a – c ), PSTHs (top row), binaural interaction matrices (middle row) and ILD-rate functions (bottom row) derived from the optimal contralateral and ipsilateral ILD response periods (black and red, respectively) from representative A1 recording sites in sham and poloxamer-injected mice. All plotting conventions are identical to those used in Fig. 4 . Note the double dissociation between disruptions of short-latency contralateral ILD sensitivity in the CHL12 unit ( b ) and long-latency ipsilateral ILD sensitivity in the CHL16 unit ( c ) compared with sham ( a ). ( d ) Slope of the linear fits applied to ILD-rate functions derived from the early contralateral (black) and late ipsilateral (red) ILD response windows ( n =127 sham units from 5 mice, 165 CHL12 units from 6 mice, 143 CHL16 units from 5 mice and 117 CHL20 units from 5 mice). ( e ) ILD associated with the highest firing rate (that is, the best ILD) based on the contralateral (black) versus ipsilateral (red) ILD response windows. All values represent mean±s.e.m. Asterisks indicate a significant difference relative to the sham group with an ANOVA after correcting for multiple comparisons ( P <0.05). Full size image To address the possibility that any stimulus feature encoded by long-latency spikes might be regulated by a developmentally delayed critical period rather than just ILD per se , we revisited the developmental regulation of aural dominance plasticity ( Fig. 3g ), only this time we separately performed the analysis on spikes occurring in the early, mid and final portion of the tone-evoked response period. Although contralateral bias decreased in later epochs of the tone-evoked response, the change was consistent for units recorded in all groups, such that the same developmental regulation of frequency tuning was observed in both early and late response periods ( Fig. 6 ). This suggests that long-latency spikes representing ipsilateral ILDs are specifically vulnerable to the effects of CHL at later ages. 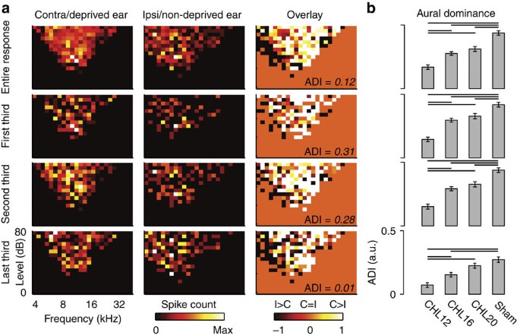Figure 6: Delayed critical period for sound features coded by long-latency spikes is specific to ILD sensitivity. (a) A1 FRAs derived from stimuli delivered separately to the contralateral/deprived (left column) and ipsilateral/non-deprived (middle column) ears in a CHL16 mouse. Aural dominance, quantified as the ratio of contralateral/ipsilateral firing rates for all tone combinations contained within the union of the two receptive fields is provided in the right column, where a more positive aural dominance index (ADI) reflects contralateral dominance in the mean of all ratio values. The overall aural dominance captured across the entire post-stimulus spiking response period (top row) can be attributed to a strong contralateral bias in the first and middle third of the response period (second and third rows, respectively) and a more balanced contralateral and ipsilateral response strength in the final portion of each response period (bottom row). (b) When aural dominance is analysed for all recording sites with bilateral FRAs (n=135 CHL12 units from 6 mice, 127 CHL16 units from 5 mice, 127 CHL20 units from 5 mice and 77 sham units from 5 mice), it is evident that although contralateral dominance may lessen in the final portion of the tone-evoked response period, it does so equally for sham controls and all CHL groups. Therefore, the age-dependent regulation of aural dominance effects is similar across all portions of the monaural tone-evoked spiking response, unlike the dichotomous effect of CHL on ILD sensitivity contained in early- versus late-response periods. Values represent mean±s.e.m. I, ipsilateral; C, contralateral. Horizontal lines indicate a significant difference between two groups after correcting for multiple comparisons (ANOVApost-hocpairwise comparisons,P<0.05). Figure 6: Delayed critical period for sound features coded by long-latency spikes is specific to ILD sensitivity. ( a ) A1 FRAs derived from stimuli delivered separately to the contralateral/deprived (left column) and ipsilateral/non-deprived (middle column) ears in a CHL16 mouse. Aural dominance, quantified as the ratio of contralateral/ipsilateral firing rates for all tone combinations contained within the union of the two receptive fields is provided in the right column, where a more positive aural dominance index (ADI) reflects contralateral dominance in the mean of all ratio values. The overall aural dominance captured across the entire post-stimulus spiking response period (top row) can be attributed to a strong contralateral bias in the first and middle third of the response period (second and third rows, respectively) and a more balanced contralateral and ipsilateral response strength in the final portion of each response period (bottom row). ( b ) When aural dominance is analysed for all recording sites with bilateral FRAs ( n =135 CHL12 units from 6 mice, 127 CHL16 units from 5 mice, 127 CHL20 units from 5 mice and 77 sham units from 5 mice), it is evident that although contralateral dominance may lessen in the final portion of the tone-evoked response period, it does so equally for sham controls and all CHL groups. Therefore, the age-dependent regulation of aural dominance effects is similar across all portions of the monaural tone-evoked spiking response, unlike the dichotomous effect of CHL on ILD sensitivity contained in early- versus late-response periods. Values represent mean±s.e.m. I, ipsilateral; C, contralateral. Horizontal lines indicate a significant difference between two groups after correcting for multiple comparisons (ANOVA post-hoc pairwise comparisons, P <0.05). Full size image A1 binaural response properties were fairly mature at the onset of hearing. The preferred frequency for each ear was closely aligned ( Fig. 1e ) and the contralateral bias in response threshold was similar to adults ( Fig. 1f ). A marked elaboration of BF range and a steep decline in response thresholds were noted between P10 and P14 ( Fig. 1b,c ), but these changes could be accounted for by ongoing cochlear maturation ( Fig. 1d ). We also noted robust ‘ EI- like’ ILD sensitivity in short-latency spikes at the onset of hearing that was qualitatively similar to recordings in older mice ( Fig. 4a,c ), in keeping with previous reports of well-defined ILD sensitivity shortly after the onset of hearing in cats and bats [35] , [36] . The precocious maturation of binaural sensitivity is likely to arise from the substantial refinement of brainstem binaural circuits that is known to occur before the onset of hearing [40] , [41] , [42] , [43] , [44] , [45] . However, by utilizing a brute force search algorithm that scanned the post-stimulus response period for spike epochs that were optimally sensitive to both contralateral and ipsilateral ILDs, we noted the delayed maturation of a long-latency response period containing fewer spikes that were nevertheless clearly associated with ipsilateral ILDs. Ipsilateral ILD sensitivity was absent at the onset of hearing ( Fig. 4b ) but came online rapidly, reaching its peak by P15–P16 ( Fig. 4d,f ). One hypothesis is that the delayed maturation of ipsilateral ILD sensitivity in long-latency spikes might be traced to the development of intracortical inhibition, which is thought to feature a more protracted development than excitation [8] , [46] (also see ref. 47 ). Auditory deprivation has been shown to interrupt the progressive reduction in inhibitory response duration that normally occurs in the early postnatal period [46] , [48] , [49] . Thus, long-latency responses to weak, delayed inputs (such as ipsilateral ILDs) may emerge only when intracortical inhibition has contracted to its mature duration, but not when inhibition is abnormally prolonged, as would occur at hearing onset [50] or following hearing loss [6] . The validity of this hypothesis remains to be tested with in vivo whole-cell recording, which offers the advantage of relating ILD spike tuning to the underlying interactions between synaptic excitation and inhibition [51] . Looking beyond underlying mechanisms, a multiplexed code for ILD sensitivity could greatly increase the bandwidth for representing binaural sound properties. With this strategy, units could dynamically encode multiple combinations of ILD and mean binaural level (rather than a single fixed property) according to when spikes occur during the post-stimulus period, as has been suggested for both spectral [38] , [52] and binaural localization cues [37] , [38] , [39] . Although many aspects of binaural sound representations were adult-like at the onset of hearing, the maintenance of these response properties was strongly disrupted by early experience with imbalanced binaural cues. Transient hearing loss in the contralateral ear was associated with elevated thresholds ( Fig. 3b ), enhanced sensitivity to the non-deprived ear ( Fig. 3b ), elevated spontaneous firing rates ( Fig. 3c ), decreased precision of interaural FRA coregistration ( Fig. 3d–f ) and reduced contralateral dominance in tone-evoked response rates ( Fig. 3g ). Other than the elevation of contralateral response threshold at P16 and comparatively weak shifts in aural dominance at both P16 and P20, reorganization of interaural frequency tuning was only observed when CHL was initiated at P12. By contrast, unilateral deprivation at P12 had comparatively weak effects on ILD tuning that were limited to short-latency spikes encoding contralateral ILDs ( Fig. 5b ). However, long-latency sensitivity to ipsilateral ILDs was strongly disrupted when CHL was introduced at P16, but not at P12 or P20, the same day ipsilateral ILD selectivity reached its maximal level in normative development ( Fig. 5c,e ). A previous study from our group described a dramatic change in contralateral and ipsilateral frequency tuning accompanied by a categorical remodelling of ILD sensitivity following reversible ear canal ligation in rats [15] . The findings reported here are similar in kind, although comparatively subtle in degree. We attribute this difference to the fact that CHL associated with poloxamer injection was less severe than ear canal ligation (an average of 15–20 dB here versus 30 dB in the previous study), the period of deprivation was far shorter (~7 days here versus 60 days in the previous study), and the post-CHL recovery time before neurophysiological recordings was longer (~7 days here versus several hours in the previous study). The outcome of our original study motivated us to more precisely probe the developmental regulation of enduring plasticity effects stemming from mild CHL that resembled a bout of otitis media in human infants. We would argue that these two studies provide a reasonable upper and lower bound on the magnitude of cortical plasticity effects associated with reversible unilateral CHL in early life, although the precise timing of developmental vulnerability to CHL will likely depend upon the species, severity and duration of hearing loss. Spatial hearing arises from three redundant acoustic cues: ILD, interaural time differences and monaural spectral cues (although the salience of each cue will vary between species according to factors such as head size, hearing range and outer ear shape). When one cue is devalued, adult humans and ferrets learn to adaptively reweight information from other cues or remap the correspondence between the altered cues and spatial locations. For instance, with several consecutive days of practice, adult ferrets or humans outfitted with a monaural earplug can learn to shift their sensitivity to other cues and eventually recover normal azimuthal localization accuracy [53] , [54] . Juvenile ferrets reared with an intermittent unilateral earplug develop a bistable neural and behavioural representation of sound location that adaptively switches between emphasizing spectral cues through the unplugged ear or dichotic cues during periods when both ears are unobstructed [55] . Similarly, adult human subjects learn over a several week period to accurately localize sound sources along the elevation axis when the spectral localization cues naturally provided by the geometry of their own outer ears are exchanged for a new set of spectral cues from foreign ears [56] . Whereas the adult nervous system is able to flexibly and adaptively reweight binaural cues according to the listening demands imposed by the particular environment, chronic experience with consistently impoverished localization cues in early life can have a lasting and negative impact on binaural hearing. Mammals reared with monaural ear plugs exhibit persistent binaural hearing deficits when tested later in life, after their hearing is audiometrically normal [57] , [58] . Similarly, humans born with unilateral ear canal malformations that are surgically repaired in later life exhibit a subnormal ability to make use of binaural cues, where the degree of behavioural deficit is positively correlated with their age at the time of corrective surgery [59] , [60] . Persistent binaural hearing deficits are far more common in instances where CHL accompanies otitis media in early childhood. According to pediatric audiology studies and the latest US census data, ~12% of children (or 2.6 million children in the United States alone) will experience at least one bout of otitis media severe enough to cause a brief, mild CHL (>25 dBHL) before reaching 5 years of age [17] , [18] . These children are at far greater risk to develop amblyaudia in later life than children who have otitis media that is not severe enough to introduce a CHL [18] . Individuals that fall under the amblyaudia spectrum exhibit reduced binaural release from masking [61] , [62] , abnormally poor sound localization accuracy [63] and deficits in complex spectrotemporal processing [64] that persist for years after the peripheral hearing loss has been resolved. Paradoxically, plasticity of binaural circuits in the auditory cortex may be both the cause of irregular binaural sound encoding during development as well as its most likely source of remediation in later life. Substantial behavioural and neural improvements in discriminating subtle differences in sound localization cues have been reported after several days of perceptual training in rodents and humans [65] , [66] . The lifelong plasticity of the adult auditory cortex is thought to be essential for the ability of mammals to gradually adapt to disordered binaural cues as pharmacological inactivation of the auditory cortex prevents the learning-induced recovery of behavioural sound localization accuracy following unilateral ear plugging [67] . Future work will be required to address the permanence of the changes described here and to establish whether applied neuroplasticity protocols in the form of auditory training or neuromodulatory pairing strategies [68] could be used to remediate suboptimal binaural sensitivity in animals, and eventually humans, recovering from impoverished auditory experience in early life. Animal preparation All procedures were approved by the Massachusetts Eye and Ear Infirmary Animal Care and Use Committee and followed the guidelines established by the National Institutes of Health for the care and use of laboratory animals. A total of 78 CBA/CaJ mice of either sex were used for all experiments. The morning that a new litter of pups was first observed was designated as postnatal day P0. Mice were anaesthetized with ketamine and xylazine for all experiments involving physiological measurements (induction with 80 mg kg −1 ketamine and 16 mg kg −1 xylazine; 45 mg kg −1 maintenance doses of ketamine, as needed). Mice were anaesthetized with isoflurane (5% induction, 1.5–2.5% maintenance in oxygen) for cases where manipulations or inspections of the ear were performed without physiological measurements. For all procedures, mice were placed atop a homeothermic blanket system with skin temperature maintained at 36.5 °C and the head immobilized with a modified head-holder. All experiments were performed inside a sound-attenuating chamber. Acoustic assemblies consisted of two miniature dynamic earphones used as sound sources and an electret condenser microphone coupled to a probe tube to measure sound pressure near the eardrum. For terminal recording procedures, the external ear was severed at the tympanic ring. The tip of each sound delivery tube was positioned against the tympanic ring and calibrated before each experiment. In P10–11 mice, care was taken to separate the meatus from the tympanic membrane to create a direct path for the acoustic stimulus. A lumen had formed in the external meatus by P12; thus, this step was unnecessary. Middle ear poloxamer hydrogel injection A slit was made in the left tragus to allow better visualization of the tympanic membrane. A small hole was made in the pars flaccida to permit the outflow of excess solution. Borosilicate glass capillary tubing was pulled to a fine, tapering point (~15 μm) and the blunt end fixed to a syringe infusion set. The syringe contained a 20% (w/w) solution of poloxamer 407 (Spectrum Chemicals) and blue dye (FD&C Blue 1) dissolved in double deionized water. The solution was prepared immediately before use and maintained at ~5 °C up to the point of injection. The injection pipette was secured within a three-dimensional micropositioner and the pipette tip advanced through the posterior quadrant of the pars tensa . Approximately 5 μl of poloxamer solution was injected under visual inspection through an operating microscope until blue fluid had filled the middle-ear cavity. Excess solution was quickly removed with an absorbent point before it transitioned to a gel. Injections were made on two successive days beginning on P12, P16 or P20. For the sham procedure, the mouse was anaesthetized at one of the ages listed above and the tragus was snipped. The middle ear was left intact owing to concerns that tympanic membrane puncture, on its own, was a form of CHL as well as a portal for middle ear infection. Otoacoustic emission measurement The probe-tube microphone was calibrated in a small coupler with a 1/8′ condenser microphone. Stimuli were generated digitally, and sound pressure was amplified and digitally sampled at 5 μs. Two tones with different carrier frequencies were delivered through the earphones. The frequencies were kept at a constant ratio ( f 2 / f 1 =1.2), and the f 2 primary was presented at 10 dB below the f 1 level. The resultant DPOAE was measured at the 2 f 1 − f 2 frequency. Each ear canal SPL measurement was obtained from 1.6 s of spectral and waveform averaging. DPOAEs were measured at five probe frequencies ( f 2 =8–32 kHz in 0.5 octave intervals) and 13 levels ( f 2 =20–80 dB SPL in 5 dB increments). The acoustic noise floor was measured at frequencies straddling the DPOAE frequency in the spectrum average. DPOAE threshold was defined as the lowest of at least two contiguous f 2 levels for which the DPOAE amplitude was at least 3 dB greater than the noise floor. ABR measurement Subdermal needle electrodes (Grass) were inserted into the ventral aspect of each pinna and a ground electrode at the base of the tail. ABRs were bandpass filtered (0.3–3 kHz), amplified 10,000 × (Grass) and sampled by the A/D board at 100 kHz. ABR was measured with tone bursts (5 ms duration, 0.5 ms onset/offset gates, 30 Hz repetition rate) at 8, 16 and 32 kHz (chronic experiments) or 16 kHz (acute experiments). Stimulus level was varied from 20–80 dB SPL, initially in 5-dB steps but increasing to 10-dB steps after a criterion response amplitude was reached (0.55 mV peak-to-peak). Stimuli were presented in opposite-polarity pairs to attenuate the contribution of microphonic potentials to the ABR waveforms. ABRs were averaged from 512 stimulus pairs (or 256 in the event the criterion response amplitude had been reached). Wave 1 threshold was defined for each stimulus type based on visual inspection of the stacked ABR waveforms. Threshold was defined as the lowest sound level that could reliably produce a stimulus-evoked peak that followed the progressive trend for decreasing amplitude and increasing latency across the full range of sound levels. Cortical unit recordings A craniotomy was made over the right auditory cortex and the brain surface was covered with high viscosity silicone oil. The dura mater was left intact. Recordings were made from the middle layers of A1 with a 4-shank 16-channel silicon probe (177 μm 2 contact area, 50 μm contact separation, 4 contacts per shank, 125 μm separation between shanks; NeuroNexus Technologies). A1 was distinguished from other cortical fields on the basis of cranial landmarks and a low-to-high, caudal-to-rostral tonotopic organization [69] , [70] . One to four separate penetrations were made per mouse. Raw signals were digitized at 32 bit and bandpass filtered at 300–5,000 Hz. High SNR multi-unit spikes were detected using an adaptive threshold set to 4.5–6 s.d. above the mean of a 5 s running average (OpenEx, Tucker-Davis Technologies). For each penetration, FRAs were derived from tone pips (50 ms duration, 4 ms raised cosine ramps, 4–45.5 kHz in 0.15 octave steps, across a maximum range of 0–90 dB SPL, interleaved and randomized for each ear, repeated twice) delivered independently to each ear (700 ms stimulus onset asynchrony). ILD sensitivity was measured from the unit responses to 45 dichotic white noise bursts of varying contralateral and ipsilateral level (100 ms duration, 5 ms raised cosine ramps, 15 repetitions). Contralateral and ipsilateral sound levels ranged from the minimum response threshold to 20 dB above threshold (5 dB steps) with ILDs spanning −20 to 20 dB (5 dB steps). To estimate the level of acoustic attenuation provided by the head, we performed extracellular unit recordings from the left and right central nucleus of the inferior colliculus using the same methods for anaesthesia, sound delivery and neurophysiological recordings described above. Before recording, the right stapes was removed and the cochlear fluids were drained, thereby inducing complete unilateral hearing loss. Sound delivery tubes were then positioned against each tympanic ring ( Fig. 7a–d ). Tones and white noise bursts were presented to the intact or destroyed ear. 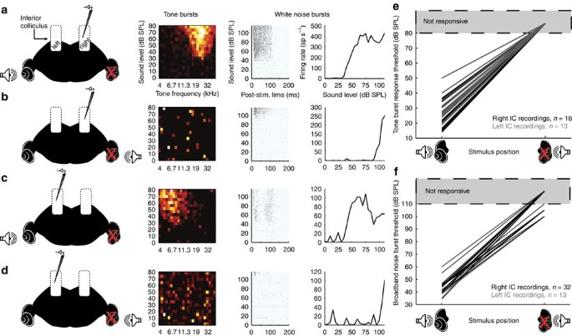Figure 7: FRA and ILD measurements are not contaminated by the contralateral transfer of acoustic energy across the head. (a–d) Extracellular unit recordings were made from the right (a,b) and left (c,d) central nucleus of the inferior colliculus after the right cochlea had been destroyed. Sound delivery tubes were positioned against the tympanic ring of the left and right ears, per normal. Example FRAs (second column), spike rastergrams (third column) and rate-level functions (fourth column) for individual recordings corresponding to the electrode and stimulus configuration depicted in the first column. Rastergrams and rate-level functions are derived from 100 ms white noise bursts. (e,f) minimum thresholds for responses evoked by tones (e) and noise bursts (f) are displayed for sounds delivered to the intact (left) and cochlectomized (right) ears. Unit responses for white noise stimuli presented to the cochlectomized ear could be elicited in 69% of the recordings but the threshold shift was far greater than the maximum ILD used inFigs 4and5(n=45 units, 61.6±0.71 dB, mean±s.e.m.). Figure 7: FRA and ILD measurements are not contaminated by the contralateral transfer of acoustic energy across the head. ( a – d ) Extracellular unit recordings were made from the right ( a , b ) and left ( c , d ) central nucleus of the inferior colliculus after the right cochlea had been destroyed. Sound delivery tubes were positioned against the tympanic ring of the left and right ears, per normal. Example FRAs (second column), spike rastergrams (third column) and rate-level functions (fourth column) for individual recordings corresponding to the electrode and stimulus configuration depicted in the first column. Rastergrams and rate-level functions are derived from 100 ms white noise bursts. ( e , f ) minimum thresholds for responses evoked by tones ( e ) and noise bursts ( f ) are displayed for sounds delivered to the intact (left) and cochlectomized (right) ears. Unit responses for white noise stimuli presented to the cochlectomized ear could be elicited in 69% of the recordings but the threshold shift was far greater than the maximum ILD used in Figs 4 and 5 ( n =45 units, 61.6±0.71 dB, mean±s.e.m.). Full size image We were unable to elicit a response from tone bursts presented to the cochlectomized ear at any frequency up to 80 dB SPL, thereby assuring that tonal receptive fields were faithful to the stimulated ear ( Fig. 7e ). Noise bursts delivered to the cochlectomized ear could drive 69% of the recorded units with thresholds that were elevated by 61.6±0.71 dB ( n =45, mean±s.e.m.) above the same unit’s sensitivity to stimulation of the intact cochlea ( Fig. 7f ). Our analysis of noise-evoked responses was restricted to stimuli with ILDs of±20 dB and mean binaural levels between threshold to 20 dB above threshold (that is, for a unit with a mean binaural threshold at 60 dB SPL, we presented noise bursts to the contralateral and ipsilateral ears ranging from 50 to 90 dB SPL as illustrated in Fig. 4a ). With this approach, the most intense sound presented would be only 30 dB above the response threshold, which is less than half of the mean threshold for activating the contralateral cochlea via cross-talk. Therefore, the neural responses presented here can be attributed to the ear that was directly stimulated. Analysis of cortical unit recordings The FRA was first smoothed by a 3 × 3 point median filter, then the spike counts were summed across sound frequencies or sound levels to create spike-frequency or spike-level functions, each of which were subsequently smoothed again with a five-point median filter. The spike-frequency function was inverted (to create a V-shape) and the tip set at the minimum threshold, defined as the inflection point on the spike-level function. FRA BF was defined as the frequency associated with the greatest number of spikes within the tone-evoked response period. The aural dominance index was defined in sites with bilateral FRAs as the mean ratio of contralateral versus ipsilateral firing rates separately defined for each frequency-level combination contained within the union of the contralateral and ipsilateral FRAs. Receptive field overlap was defined as the number of frequency–intensity points contained within the intersection of the contralateral and ipsilateral FRAs divided by the number of points contained within their union. The developmental analysis was based on 1,262 unit recordings in 35 mice, of which 1,001 units were responsive to ipsilateral or contralateral sound (P10, n =3/3 (recording sites/animals); P11, n =55/3; P12, n =70/3; P13, n =42/3; P14, n =96/4; P15, n =107/3; P16, n =91/3; P17, n =162/4; adult (8–14 weeks) n =375/9). The effects of hearing loss were based on 612 units in 21 mice (Sham, n =142/5; CHL12, n =163/6, CHL16, n =159/5 and CHL20, n =148/5). For dichotic noise burst stimuli, analysis was restricted to recording sites that yielded a FRA for either the contralateral or ipsilateral ear, were significantly driven by dichotic white noise bursts (unpaired Student’s t -test of pre- versus post-stimulus spike rates for all stimulus combinations, P <0.001) and had a minimum response threshold for average binaural sound levels ≤75 dB SPL ( n =610 and 552 recordings sites for the developmental study and plasticity study, respectively). Minimum threshold was defined at each recording site as the lowest mean binaural level for which the firing rate of at least one ILD combination was more than 3.5 s.d. above its spontaneous firing rate. The timing of the overall noise-evoked response period were the first and last bins of a contiguous response period containing firing rates at least 4 s.d. above the spontaneous rate. We separately quantified response periods containing spikes evoked by contralateral versus ipsilateral ILDs. The timing of each window was determined by measuring when spiking activity for the 20 contralateral ILDs (ILD=5 to 20 dB at 5 mean binaural levels) was most different from the 20 ipsilateral ILD combinations (ILD=−5 to −20 dB at 5 mean binaural levels), respectively. As the precise timing of response periods containing spikes evoked by contralateral versus ipsilateral ILDs might vary across development between hearing loss conditions, or between different units, the onset and offset windows that captured the strongest contralateral and ipsilateral ILD sensitivity were left as free parameters to be determined by a brute force exhaustive search approach. The search algorithm was limited by three constraints: first, the onset of contralateral and ipsilateral ILD response windows must both be contained within the entire response period; second, the windows must avoid offset responses by terminating <100 ms from the onset response; finally, each window must be at least 20 ms in duration. This approach allowed us to objectively determine the post-stimulus response windows that maximized the difference in mean firing rate evoked by contralateral versus ipsilateral ILDs without making any assumptions as to when these responses occurred. Once the timing of each response window was established, the mean rate-ILD functions were constructed from the five binaural levels ranging from threshold to 20 dB above threshold. ILD sensitivity was quantified by calculating the slope of the linear fit applied to the mean ILD function. How to cite this article: Polley, D. B. et al . Brief hearing loss disrupts binaural integration during two early critical periods of auditory cortex development. Nat. Commun. 4:2547 doi: 10.1038/ncomms3547 (2013).